Structural characterization of the substrate transfer mechanism in Hsp70/Hsp90 folding machinery mediated by Hop In eukarya, chaperones Hsp70 and Hsp90 act coordinately in the folding and maturation of a range of key proteins with the help of several co-chaperones, especially Hop. Although biochemical data define the Hop-mediated Hsp70–Hsp90 substrate transfer mechanism, the intrinsic flexibility of these proteins and the dynamic nature of their complexes have limited the structural studies of this mechanism. Here we generate several complexes in the Hsp70/Hsp90 folding pathway (Hsp90:Hop, Hsp90:Hop:Hsp70 and Hsp90:Hop:Hsp70 with a fragment of the client protein glucocorticoid receptor (GR-LBD)), and determine their 3D structure using electron microscopy techniques. Our results show that one Hop molecule binds to one side of the Hsp90 dimer in both extended and compact conformations, through Hop domain rearrangement that take place when Hsp70 or Hsp70:GR-LBD bind to Hsp90:Hop. The compact conformation of the Hsp90:Hop:Hsp70:GR-LBD complex shows that GR-LBD binds to the side of the Hsp90 dimer opposite the Hop attachment site. Hsp70 and Hsp90 are the most abundant chaperones and have important roles in quality control of cell protein [1] . The Hsp70s have been characterized extensively; they bind and release substrates using an ATP-dependent mechanism regulated by allosteric interactions between the two Hsp70 domains, the amino-terminal (N-terminal) nucleotide-binding domain (Hsp70 NBD ) and the carboxyl-terminal (C-terminal) substrate-binding domain (Hsp70 SBD ) [2] , [3] , which are connected by a highly conserved linker [4] ( Supplementary Fig. 1a ). The Hsp90 are dimeric proteins; each monomer is composed of three domains, the N-terminal domain (Hsp90-N) with the ATP-binding site, the middle domain (Hsp90-M), the main region responsible for substrate:protein interactions and the C-terminal domain (Hsp90-C), which hosts the dimerization site [5] ( Supplementary Fig. 1b ). Hsp90 is a highly flexible molecule and adopts distinct conformations during its functional cycle, which is regulated in turn by a variety of cofactors [3] , [6] , [7] , [8] , [9] , as is also the case for Hsp70 (ref. 3 ). Hsp70 and Hsp90 not only have important roles as primary chaperones but also cooperate in targeting clients for folding, assembly and maturation of a broad range of quasi-native substrates, termed client proteins, such as transcription factors, kinases and nuclear receptors like the steroid hormone receptors (SHR) [10] , [11] . These processes are aided by various co-chaperones [12] , one of the best studied of which is the Hsp70–Hsp90-organizing protein (Hop; Sti1 in yeast) [13] , a monomer [14] composed of three tetratricopeptide repeat domains (TPR1, TPR2A, TPR2B) involved in protein–protein interaction, and two small aspartic acid–proline repeat domains (DP1, DP2) involved in client activation [15] , [16] ( Supplementary Fig. 1c ). A flexible linker connects two Hop modules, a TPR1-DP1 module that participates for substrate transfer, and a TPR2A-TPR2B-DP2 module, in which the TPR2A and TPR2B domains work as a rigid body, proposed to be the active core of the protein [16] ( Supplementary Fig. 1c ). All TPR interact specifically with Hsp70 or Hsp90 C-terminal sequences; TPR2A binds preferentially to Hsp90, whereas TPR1 and TPR2B bind to Hsp70 (refs 16 , 17 ). Secondary Hop interactions are nonetheless TPR independent [18] , [19] . The concerted action of Hsp70 and Hsp90 in the maturation of certain client proteins such as SHR has been characterized in part [20] , [21] , [22] , and is initiated by SHR binding to Hsp70 (refs 23 , 24 ). The receptor is then transferred to Hsp90 via a preformed Hsp90:Hop complex, to form a Hsp70:Hop:Hsp90:SHR complex termed ‘foldosome’ [13] , [21] . Subsequent interaction with other co-chaperones such as PPIase or p23 (refs 20 , 25 ) generates a Hsp90:SHR complex in which Hsp90 folds the ligand-binding pocket of the SHR, leading to a hormone-binding-competent conformation [26] , [27] . Despite exhaustive biochemical characterization of the Hsp70/Hsp90 machinery, little is known about the structural features of these intermediate complexes, due to the intrinsic flexibility of their components and their highly dynamic behaviour. In this study, we generate several of the complexes formed in the Hsp70/Hsp90 folding pathway and determined their three-dimensional (3D) structure using electron microscopy (EM) and image processing. Our results indicate that one Hop molecule binds to the Hsp90 dimer and through domain rearrangement, gives rise to two main conformations, an extended structure that recognizes and interacts with Hsp70, and a compact one in which Hsp70 is in contact with one Hsp90 monomer. Movement between these two modes delivers the Hsp70-bound substrate to the side of the Hsp90 dimer opposite the site of Hop binding. These findings pave the way for a deeper understanding of the structural aspects of the Hsp70/Hsp90 folding machinery. Structure of the Hsp90:Hop complex In a first step to structurally characterize the Hsp70/Hsp90 folding machinery, we formed and purified the Hsp90:Hop complex in various conditions (no nucleotide, with ADP or ATP). The best results were obtained with ADP as described [21] . We purified the complex by gel filtration chromatography, but it separated poorly from the Hsp90 dimer and was highly heterogeneous, as seen by EM and reported by others [28] . We thus used GraFix [29] , a gradient technique for purifying and stabilizing macromolecular complexes using low-level glutaraldehyde, which is particularly suitable for EM ( Supplementary Fig. 2a ); thus treated, Hsp90:Hop was homogeneous as judged by EM. We classified 21,003 particles of the negatively stained complex, and found a certain degree of heterogeneity (see below), but the largest population was used to generate a 3D reconstruction of the Hsp90:Hop complex (21 Å resolution; see Methods and Supplementary Fig. 3 ). The complex has a triangular shape of 130 × 110 × 80 Å ( Fig. 1a ). A control gradient without crosslinker yielded a more heterogeneous sample, although the largest population generated structures resembling those obtained with crosslinking ( Supplementary Fig. 4a ). Reconstruction of the GraFix-purified complex gave similar results with or without molybdate, used to avoid autoproteolysis and to stabilize the complex ( Supplementary Fig. 4c ). 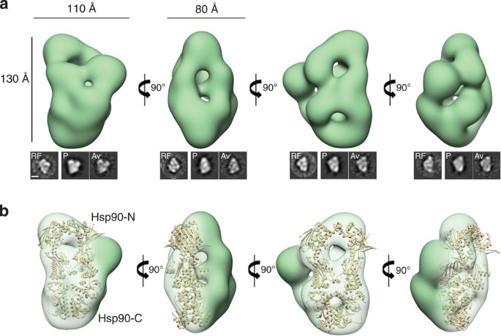Figure 1: 3D reconstruction of the Hsp90:Hop complex. (a) Top, four orthogonal views of the Hsp90:Hop complex 3D reconstruction (21 Å resolution). The same four views will be used in subsequent figures. Bottom, reference-free (RF) class averages, projections (P) and 2D averages (Av) of the final model, shown in the same orientations as at the top. Scale bar, 50 Å. (b) Docking of a modified Hsp90·ADP atomic structure (pdb 2IOP) into the 3D reconstruction of the Hsp90:Hop complex. The dark green area is assigned to Hop. Figure 1: 3D reconstruction of the Hsp90:Hop complex. ( a ) Top, four orthogonal views of the Hsp90:Hop complex 3D reconstruction (21 Å resolution). The same four views will be used in subsequent figures. Bottom, reference-free (RF) class averages, projections (P) and 2D averages (Av) of the final model, shown in the same orientations as at the top. Scale bar, 50 Å. ( b ) Docking of a modified Hsp90·ADP atomic structure (pdb 2IOP) into the 3D reconstruction of the Hsp90:Hop complex. The dark green area is assigned to Hop. Full size image The location of the Hsp90 dimer (ADP conformation) within the volume of the complex is unequivocal ( Fig. 1b ); Hsp90 can only be placed in one side of the reconstructed volume, with Hsp90-C located in the narrow part of the reconstructed structure. When we use the atomic structure of the semiclosed, ADP conformation [8] , the fit of Hsp90 into the 3D reconstruction of the Hsp90:Hop complex is particularly good. As a control, we carried out a structural analysis of the Hsp90 dimer with ADP. The sample was negatively stained; EM analysis showed dimeric Hsp90 particles ( Supplementary Fig. 5a ). We processed 12,997 particles, which indicated that most variability was confined to the Hsp90-N domains ( Supplementary Fig. 5b ). Both the two-dimensional (2D) analysis and the 3D reconstruction of the largest population ( Supplementary Fig. 5c ) pointed to an Hsp90 dimer in a semiclosed conformation, similar to the Hsp90 atomic structure (ADP) [8] . The unassigned mass of the Hsp90:Hop complex indicated only a single Hop monomer, a result reinforced by the asymmetry of the volume. Although we visualized five masses corresponding to the five Hop domains, we could not assign them directly due to the low resolution of the 3D reconstruction and thus applied alternative approaches. We first localized the DP2 domain by immunomicroscopy, using a domain-specific monoclonal antibody ( Fig. 2a ). Aliquots of the purified immunocomplex were stained and analysed by EM, which showed an apparently homogeneous population. A total of 13,259 particles were processed; comparison of one of the most common 2D views of the immunocomplex with the same view of the Hsp90:Hop complex clearly indicated an extra mass ( Fig. 2b , arrow). The 3D reconstruction of the immunocomplex (35 Å resolution; Fig. 2c ) showed, in addition to the triangular Hsp90:Hop complex, a V-shaped mass assigned to the antibody ( Fig. 2d ). Both antibody arms contact the Hsp90:Hop complex, but only one interacts with an unassigned mass, which we assigned to the DP2 domain, whose atomic structure [16] fits well into this part of the volume ( Fig. 2d ). 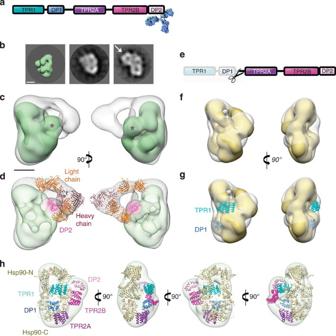Figure 2: Hop domain localization in the Hsp90:Hop complex. (a) Scheme of the Hop domains showing the immunolabel of the DP2 domain. (b) Comparison of the Hsp90:Hop complex 3D reconstruction (left) with its 2D average (centre) and the same view of the Hsp90:Hop:anti-DP2 immunocomplex (right). The arrow indicates the position of the anti-DP2 monoclonal antibody. Scale bar, 50 Å. (c) Two orthogonal views of the Hsp90:Hop complex 3D reconstructions (green) superimposed on the Hsp90:Hop:anti-DP2 immunocomplex (white). The top arm of the antibody interacts with the region assigned to the Hsp90 dimer. The bottom arm interacts with a region assigned to Hop (asterisk). (d) Docking of the atomic structures of an antibody molecule (pdb 1IGY) and the DP2 domain (pdb 2LLW) into the volumes shown inc. (e) Scheme of the Δ(TPR1-DP1)Hop mutant, which lacks TPR1 and DP1 domains. (f) Two orthogonal views of the Hsp90:Hop complex 3D reconstruction (grey, transparent) superimposed on Hsp90:Δ(TPR1-DP1)Hop complex (yellow, solid). (g) Docking of the atomic structure of the TPR1 and DP1 domains (pdb 1ELLW and 2LLV, respectively) into the mass of the Hsp90:Hop complex absent in the Hsp90: Δ(TPR1-DP1)Hop complex. (h) The same orthogonal views of the Hsp90:Hop complex as inFig. 1a), with the atomic structures of Hsp90 (pdb 2IOP) and the Hop domains TPR1 (pdb 1ELW), DP1 (pdb 2LLV), the TPR2A-TPR2B module (pdb3UQ3) and DP2 (pdb (2LLW). Colour coded as ina. Scale bar incindicates 50 Å for all the volumes of the figure. Figure 2: Hop domain localization in the Hsp90:Hop complex. ( a ) Scheme of the Hop domains showing the immunolabel of the DP2 domain. ( b ) Comparison of the Hsp90:Hop complex 3D reconstruction (left) with its 2D average (centre) and the same view of the Hsp90:Hop:anti-DP2 immunocomplex (right). The arrow indicates the position of the anti-DP2 monoclonal antibody. Scale bar, 50 Å. ( c ) Two orthogonal views of the Hsp90:Hop complex 3D reconstructions (green) superimposed on the Hsp90:Hop:anti-DP2 immunocomplex (white). The top arm of the antibody interacts with the region assigned to the Hsp90 dimer. The bottom arm interacts with a region assigned to Hop (asterisk). ( d ) Docking of the atomic structures of an antibody molecule (pdb 1IGY) and the DP2 domain (pdb 2LLW) into the volumes shown in c . ( e ) Scheme of the Δ(TPR1-DP1)Hop mutant, which lacks TPR1 and DP1 domains. ( f ) Two orthogonal views of the Hsp90:Hop complex 3D reconstruction (grey, transparent) superimposed on Hsp90:Δ(TPR1-DP1)Hop complex (yellow, solid). ( g ) Docking of the atomic structure of the TPR1 and DP1 domains (pdb 1ELLW and 2LLV, respectively) into the mass of the Hsp90:Hop complex absent in the Hsp90: Δ(TPR1-DP1)Hop complex. ( h ) The same orthogonal views of the Hsp90:Hop complex as in Fig. 1a ), with the atomic structures of Hsp90 (pdb 2IOP) and the Hop domains TPR1 (pdb 1ELW), DP1 (pdb 2LLV), the TPR2A-TPR2B module (pdb3UQ3) and DP2 (pdb (2LLW). Colour coded as in a . Scale bar in c indicates 50 Å for all the volumes of the figure. Full size image In a second approach, we localized the TPR1-DP1 domains indirectly using a Hop mutant that lacks these two domains (Δ(TPR1-DP1)Hop; Fig. 2e ). We formed the complex and analysed it by EM. The 3D reconstruction generated from 33,845 negatively stained particles (23 Å resolution; Fig. 2f ) resembled that of the Hsp90:Hop complex, except that it lacked mass in the middle of the volume. The atomic structures of TPR1 (ref. 17 ) and DP1 (ref. 16 ) dock well in the appropriate masses of the difference density map for the two volumes ( Fig. 2g ). Once TPR1, DP1 and DP2 domains were localized, placement of the central TPR2A-TPR2B module [16] in the two remaining masses is straightforward. TPR2A, which interacts with the Hsp90 C-terminal MEEVD motif, was placed near this region, and the TPR2B domain in the remaining density, was located near DP2 and interacted with Hsp90-M, as described [16] ( Fig. 2h ). These findings show a Hop monomer that interacts with one side of an Hsp90 dimer in a semiclosed conformation, with the Hop domains arranged anticlockwise and in close contact with the Hsp90-M and Hsp90-C domains ( Fig. 2h ). To determine whether this type of interaction is conserved in other eukaryotic systems, we analysed the yeast counterparts in a similar manner. We purified the yeast Hsp90:Hop(Sti1) complex in the presence of ADP, classified 18,738 negatively stained particles and used the largest population for a 3D reconstruction (25 Å resolution, Supplementary Fig. 2b ). The volume obtained was similar to its human counterpart, and the five Hop domains could be fitted in a similar manner ( Supplementary Fig. 2c ), although here a slightly more open conformation of Hsp90 docked better. These findings suggest a conserved mechanism for the Hsp90:Hop interaction, reinforced by the fact that heterologous complexes can be formed between human and yeast proteins (not shown). The heterogeneity of the crosslinked Hsp90:Hop complex was studied further. The 2D classification procedures showed that the largest difference was for a majority, compact population used for the 3D reconstruction; a minority population showed a small mass protruding from the main one ( Supplementary Fig. 4b ). Comparison of these two structures, as well as knowledge of the locations of Hop domain docking into the Hsp90:Hop structure, suggest that TPR1 and DP1 domains are those that undergo changes (see below). Structure of the Hsp90:Hop:Hsp70 complex We analysed the next step in the Hsp70/Hsp90 folding pathway, that of complex formation between Hsp90:Hop and Hsp70. As described [21] , the addition of a substoichiometric amount of Hsp40 improved the efficiency of ternary complex formation, although Hsp40 was not present in the final complex ( Supplementary Fig. 6a ). A total of 41,393 particles of the purified complex were classified (ML2D and CL2D; see Methods) to select a majority population (~80% of particles), which was used for 3D reconstruction (23 Å resolution; Fig. 3a ). The volume generated is similar to that of the binary complex, except for a small, triangular mass protruding from one vertex of the reconstructed volume, which we assigned to Hsp70. As in the case of the Hsp90:Hop complex, the Hsp90 dimer can be unequivocally placed on one side of the complex ( Fig. 3b ), with the remaining reconstructed mass assigned to Hop and Hsp70. 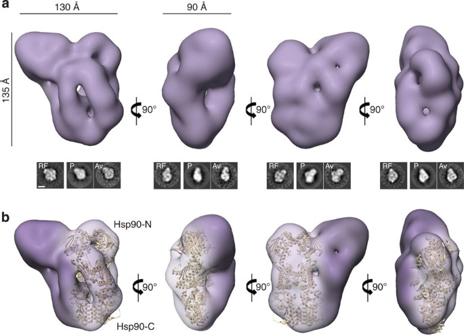Figure 3: 3D reconstruction of the Hsp90:Hop:Hsp70 complex. (a) Top, four orthogonal views of the Hsp90:Hop:Hsp70 complex 3D reconstruction (23 Å resolution). Bottom, reference-free (RF) class averages, projections (P) and 2D averages (Av) of the final model in the same orientations as at the top. Bar indicates 50 Å. (b) Docking of a modified Hsp90·ADP atomic structure (pdb 2IOP) into the Hsp90:Hop:Hsp70 complex 3D reconstruction. The dark violet area is assigned to Hop and Hsp70. Figure 3: 3D reconstruction of the Hsp90:Hop:Hsp70 complex. ( a ) Top, four orthogonal views of the Hsp90:Hop:Hsp70 complex 3D reconstruction (23 Å resolution). Bottom, reference-free (RF) class averages, projections (P) and 2D averages (Av) of the final model in the same orientations as at the top. Bar indicates 50 Å. ( b ) Docking of a modified Hsp90·ADP atomic structure (pdb 2IOP) into the Hsp90:Hop:Hsp70 complex 3D reconstruction. The dark violet area is assigned to Hop and Hsp70. Full size image We used specific monoclonal antibodies to locate the two Hsp70 domains (Hsp70 NBD , Hsp70 SBD ) by immunomicroscopy ( Fig. 4a,e ). Immunocomplexes were formed, purified using Grafix and analysed by EM, which showed heterogeneous populations for both. In the first case, we selected 19,026 negatively stained particles; 2D processing showed an extra mass, assigned to the antibody ( Fig. 4b , arrow). The 3D reconstruction of the immunocomplex (30 Å resolution; Fig. 4c ) revealed more clearly the V-shaped mass characteristic of the antibody, bound to the extra mass in the ternary complex. Docking of the atomic structure of an antibody [30] is straightforward; this, and the triangular shape of the extra mass that resembles the reported Hsp70 NBD structure [4] made its docking and location unambiguous ( Fig. 4d ). To locate Hsp70 SBD , we generated the immunocomplex with a monoclonal antibody that recognizes its C-terminal part ( Fig. 4e , top). A total of 17,790 particles were processed, and comparison of similar 2D views of the immunocomplex and the ternary complex showed an extra mass, assigned to the antibody ( Fig. 4f , red arrow). Superposition of the 3D reconstruction of the immunocomplex (25 Å resolution; Fig. 4g ) with that of the ternary complex, confirmed the extra mass, which confirmed our assignment ( Fig. 4g , star). Docking of the atomic structures of an antibody molecule [30] and Hsp70 SBD (ref. 31 ) into their corresponding masses reinforced the location of the latter. This result was confirmed by an independent experiment using the Fab fragment of the monoclonal antibody ( Fig. 4e , bottom), which binds to the same region of the Hsp90:Hop:Hsp70 complex, as seen by 2D analysis of the immunocomplex ( Fig. 4f , white arrow) or in its 3D reconstruction ( Fig. 4g ; right, star). This result strengthens our data regarding Hsp70 SBD localization in the Hsp90:Hop:Hsp70 complex. Once the Hsp90 dimer and Hsp70 were mapped into the ternary complex, the five Hop domains could be docked into their corresponding masses, as for the binary complex. 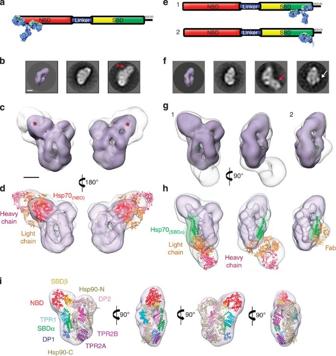Figure 4: Localization of Hsp70 and Hop domains in the Hsp90:Hop:Hsp70 complex. (a) Scheme of Hsp70 showing the immunolabel of Hsp70NBD. (b) Comparison of the Hsp90:Hop:Hsp70 complex 3D reconstruction (left) with its 2D average (centre) and that of the Hsp90:Hop:Hsp70:anti-Hsp70NBDimmunocomplex (right). The arrow indicates the anti-Hsp70NBDantibody. Bar indicates 50 Å forbandf. (c) Superposition of the 3D reconstructions of the Hsp90:Hop:Hsp70 complex (violet) and the Hsp90:Hop:Hsp70:anti-Hsp70NBDimmunocomplex (white). The two antibody arms interact with the mass assigned to Hsp70NBD(asterisk). (d) Docking of an antibody molecule (pdb 1IGY) and Hsp70NBD(pdb 1YUW) into the volumes inc. (e) Scheme of Hsp70 showing the Hsp70SBDimmunolabels, with a full-length monoclonal antibody (1) or a Fab fragment (2). (f) Comparison (left to right) of the Hsp90:Hop:Hsp70 complex 3D reconstruction (side view), the 2D KerDenSom average, the same view of the Hsp90:Hop:Hsp70:anti-Hsp70SBDimmunocomplex and that with a Fab fragment. Red arrow indicates the antibody; white arrow, Fab fragment. (g) Left and centre, two orthogonal views of the Hsp90:Hop:Hsp70 complex (violet) superimposed on the Hsp90:Hop:Hsp70:anti-Hsp70SBDimmunocomplex (white). Right, view of the superposition of the Hsp90:Hop:Hsp70 complex (violet) and the Hsp90:Hop:Hsp70:anti-Hsp70SBDimmunocomplex, in this case generated with a Fab fragment (white). The asterisks indicate the common binding site of the two immunoparticles. (h) As ing, with the docking of Hsp70αSBD(pdb 3DPO), an antibody molecule (pdb 1IGY) (left and centre), and a Fab fragment (pdb 1YEF70) (right). (i) Four orthogonal views of the Hsp90:Hop:Hsp70 complex with atomic structures of Hsp90, the Hop domains (as inFig. 2h), Hsp70NBD(pdb 1YUW) and Hsp70SBD(pdb 3DPO). Bar incindicates 50 Å for all the volumes of the figure. Figure 4: Localization of Hsp70 and Hop domains in the Hsp90:Hop:Hsp70 complex. ( a ) Scheme of Hsp70 showing the immunolabel of Hsp70 NBD . ( b ) Comparison of the Hsp90:Hop:Hsp70 complex 3D reconstruction (left) with its 2D average (centre) and that of the Hsp90:Hop:Hsp70:anti-Hsp70 NBD immunocomplex (right). The arrow indicates the anti-Hsp70 NBD antibody. Bar indicates 50 Å for b and f . ( c ) Superposition of the 3D reconstructions of the Hsp90:Hop:Hsp70 complex (violet) and the Hsp90:Hop:Hsp70:anti-Hsp70 NBD immunocomplex (white). The two antibody arms interact with the mass assigned to Hsp70 NBD (asterisk). ( d ) Docking of an antibody molecule (pdb 1IGY) and Hsp70 NBD (pdb 1YUW) into the volumes in c . ( e ) Scheme of Hsp70 showing the Hsp70 SBD immunolabels, with a full-length monoclonal antibody (1) or a Fab fragment (2). ( f ) Comparison (left to right) of the Hsp90:Hop:Hsp70 complex 3D reconstruction (side view), the 2D KerDenSom average, the same view of the Hsp90:Hop:Hsp70:anti-Hsp70 SBD immunocomplex and that with a Fab fragment. Red arrow indicates the antibody; white arrow, Fab fragment. ( g ) Left and centre, two orthogonal views of the Hsp90:Hop:Hsp70 complex (violet) superimposed on the Hsp90:Hop:Hsp70:anti-Hsp70 SBD immunocomplex (white). Right, view of the superposition of the Hsp90:Hop:Hsp70 complex (violet) and the Hsp90:Hop:Hsp70:anti-Hsp70 SBD immunocomplex, in this case generated with a Fab fragment (white). The asterisks indicate the common binding site of the two immunoparticles. ( h ) As in g , with the docking of Hsp70 αSBD (pdb 3DPO), an antibody molecule (pdb 1IGY) (left and centre), and a Fab fragment (pdb 1YEF [70] ) (right). ( i ) Four orthogonal views of the Hsp90:Hop:Hsp70 complex with atomic structures of Hsp90, the Hop domains (as in Fig. 2h ), Hsp70 NBD (pdb 1YUW) and Hsp70 SBD (pdb 3DPO). Bar in c indicates 50 Å for all the volumes of the figure. Full size image This information can be used to generate a pseudoatomic model of the Hsp90:Hop:Hsp70 complex ( Fig. 4i ), which indicates a compact structure with a single Hop molecule in close contact with one side of the Hs90 dimer. Hsp70 is located in the same side of the Hsp90 dimer as Hop, but unlike the co-chaperone, it interacts with only one of the two Hsp90 monomers. We found that the Hop-binding domain Hsp70 SBD was in close proximity to its two potential Hop-binding sites, TPR1 and TPR2B [16] . Although Hsp70 and Hsp90 are reported to interact through Hop [32] , [33] , we observed Hsp70 NBD in direct contact with the N-terminal region of one of the Hsp90 monomers ( Fig. 4i ). To determine whether the structure of the human ternary complex is conserved in other eukaryotic systems, we performed a similar study in the yeast system. We formed a ternary complex by incubating purified yeast Hsp90, Hop(Sti1), Hsp40(Ydj1) and Hsp70(Ssa1). A total of 19,768 negatively stained particles of the purified complex were classified and the largest, compact population used for 3D reconstruction (24 Å resolution; Supplementary Fig. 6b ). The volume generated was very similar to its human counterpart and allowed direct docking of the pseudoatomic model generated for the human ternary complex ( Supplementary Fig. 6c ). This indicates a conserved mechanism for the interaction between Hsp90:Hop and Hsp70. Although the arrangement of the five Hop domains appears to be maintained in the binary and ternary complexes, careful examination of the two structures shows a different picture. When the masses assigned to the Hsp90 dimer in the binary and ternary complexes were made to coincide ( Fig. 5a ), we found evident lateral movement of the Hop modules (TPR1-DP1 and TPR2A-TPR2B-DP2) after Hsp70 interaction with Hsp90:Hop ( Fig. 5b ), probably induced by Hsp70 SBD interaction with TPR2B [16] . 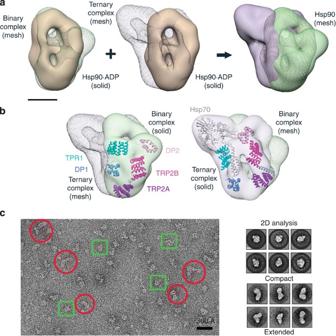Figure 5: Flexibility of the Hsp90:Hop:Hsp70 complex. (a) Location of the Hsp90 dimer in the Hsp90:Hop (left) and the Hsp90:Hop:Hsp70 complex (centre). The Hsp90 dimer 3D reconstruction (brown, solid) is docked into the binary (green, mesh) and ternary (white, mesh) complexes. Right, relative positions of the binary (green) and ternary (violet) complexes after matching the positions of the Hsp90 dimer in the two complexes. (b) Using the information generated ina, superposition of the binary and ternary complexes, with the docking of Hop domains worked out for the binary (left) and ternary (right) complexes, as shown inFigs 2hand4i, respectively. Hsp70 docking is also shown in the ternary complex (right). (c) Left, EM field of the human Hsp90:Hop:Hsp70 complex. Green squares indicate particles with a compact conformation, whereas red circles signal particles with an extended conformation. Right, various reference-free 2D averages from the two populations. Scale bar inashows 50 Å for all volumes. Figure 5: Flexibility of the Hsp90:Hop:Hsp70 complex. ( a ) Location of the Hsp90 dimer in the Hsp90:Hop (left) and the Hsp90:Hop:Hsp70 complex (centre). The Hsp90 dimer 3D reconstruction (brown, solid) is docked into the binary (green, mesh) and ternary (white, mesh) complexes. Right, relative positions of the binary (green) and ternary (violet) complexes after matching the positions of the Hsp90 dimer in the two complexes. ( b ) Using the information generated in a , superposition of the binary and ternary complexes, with the docking of Hop domains worked out for the binary (left) and ternary (right) complexes, as shown in Figs 2h and 4i , respectively. Hsp70 docking is also shown in the ternary complex (right). ( c ) Left, EM field of the human Hsp90:Hop:Hsp70 complex. Green squares indicate particles with a compact conformation, whereas red circles signal particles with an extended conformation. Right, various reference-free 2D averages from the two populations. Scale bar in a shows 50 Å for all volumes. Full size image The extended conformation of the Hsp90:Hop:Hsp70 complex As described above, the human and yeast ternary complexes are clearly heterogeneous ( Fig. 5c ); both have a majority population that can be described as ‘compact’, and a less frequent population (~15%) with a elongated ‘L’-shape formed by two asymmetric masses, which we termed ‘extended’. In the Hsp70/Hsp90 folding pathway, Hsp90:Hop is suggested to interact through Hop TPR1 with Hsp70 SBD , which is then transferred to the TPR2A-TPR2B-DP2 module for interaction with TPR2B [16] . We hypothesized that the first step might correspond to the ‘extended’ and the second, to the ‘compact’ conformations. We used two strategies to characterize the extended conformation. In the first, we selected 6,651 particles of the extended conformation from the bulk of particles selected for characterization of the human ternary complex. After extensive 2D classification, we used 3,240 highly homogeneous particles to generate a 3D reconstruction that showed two masses connected by a linker (26 Å resolution; Fig. 6a ). Docking of the atomic structure of the Hsp90 dimer (ADP conformation) was only possible in the larger mass, and is unambiguous ( Fig. 6c ). On the basis of the docking for the compact conformation and available biochemical information, we assigned the remaining volume of this larger mass to the TPR2A-TPR2B-DP2 module, with the Hsp90-binding domain TPR2A located near the linker and in close contact with the Hsp90-C dimerization domain. The smaller mass could therefore be assigned to Hsp70 and to the Hop TPR1-DP1 module, which interacts with Hsp70 SBD via TPR1. We confirmed the presence of Hsp70 in the smaller mass using an anti-Hsp70 NBD antibody ( Fig. 6b ). Finally, the linker between the masses of the reconstructed complex was assigned to the flexible, non-structured region of Hop (~60 residues) that connects the TPR1-DP1 and TPR2A-TPR2B-DP2 modules ( Fig. 6c ). 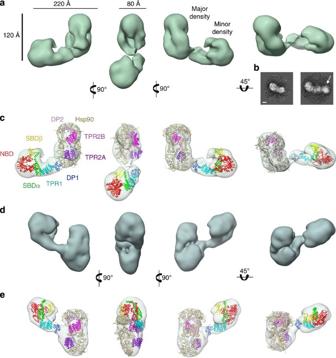Figure 6: 3D reconstructions of the extended conformation of human and yeast Hsp90:Hop:Hsp70 complexes. (a) The four standard orthogonal views of the extended conformation of the human Hsp90:Hop:Hsp90 complex. (b) Location of Hsp70 in the extended conformation of the Hsp90:Hop:Hsp70 complex. A 2D class average of the extended conformation of the Hsp90:Hop:Hsp70 complex, similar to the view of the volume of the complex shown above, ina, either in the absence (left) or presence (right) of the anti-Hsp70NBDantibody (marked with an arrow). Scale bar, 50 Å. (c) Proposed Hsp90, Hop and hsp70 domain docking in the volumes shown ina. (d) The four standard orthogonal views of the extended conformation of the yeast Hsp90:Hop(R469A):Hsp90 complex. (e) Proposed Hsp90, Hop and hsp70 domain docking in the volumes shown ind. Figure 6: 3D reconstructions of the extended conformation of human and yeast Hsp90:Hop:Hsp70 complexes. ( a ) The four standard orthogonal views of the extended conformation of the human Hsp90:Hop:Hsp90 complex. ( b ) Location of Hsp70 in the extended conformation of the Hsp90:Hop:Hsp70 complex. A 2D class average of the extended conformation of the Hsp90:Hop:Hsp70 complex, similar to the view of the volume of the complex shown above, in a , either in the absence (left) or presence (right) of the anti-Hsp70 NBD antibody (marked with an arrow). Scale bar, 50 Å. ( c ) Proposed Hsp90, Hop and hsp70 domain docking in the volumes shown in a . ( d ) The four standard orthogonal views of the extended conformation of the yeast Hsp90:Hop(R469A):Hsp90 complex. ( e ) Proposed Hsp90, Hop and hsp70 domain docking in the volumes shown in d . Full size image For the second approach, we generated a ternary complex with yeast Hsp90, Hsp70 and a yeast Hop mutant (Hop(R469A)) that blocks Hsp70 binding to TPR2B, thus favouring the extended conformation by forcing Hsp70-Hop binding only through the TPR1 domain [16] . This was confirmed when aliquots of the purified Hsp90:Hop(R469A):Hsp70 complex were stained and observed by EM, as 40% of the particles could be classified as an extended conformation. We processed 8,849 particles of the extended conformation to generate a 3D reconstruction ( Fig. 6d ), which again showed two unequal masses connected by a linker. In this case, the degree of aperture was smaller, and intermediate between the more open conformation of the human extended complex and the compact conformation of the human and yeast complexes (compare Fig. 6a,d ). As for the human extended conformation, the Hsp90 dimer could only be docked in the larger of the two masses, leaving space for the TPR2A-TPR2B-DP2 module. The smaller mass is therefore assigned to Hsp70 and the Hop TPR1-DP1 module ( Fig. 6e ). These results clearly indicate the existence of an extended conformation and provide a structural basis for two distinct Hsp90:Hop:Hsp70 complex modes due to Hop flexibility. The fact that extended and compact conformations are observed in man and yeast again points to a shared mechanism in the Hsp70/Hsp90 folding pathway. To confirm that there are indeed two conformations in the ternary complex, we used analytical ultracentrifugation in the same conditions applied for EM samples, without the crosslinker ( Supplementary Fig. 7c ). Of the five peaks in the sedimentation profile, the peak with the lowest s -value was assigned to free monomeric Hsp70; the second lowest might be assigned to dimeric Hsp70 or to the Hsp70:Hop complex [16] , [34] , [35] , [36] ( Supplementary Fig. 7a ). The central peak had an s -value similar to that of the Hsp90:Hop complex ( Supplementary Fig. 7b ), to which it was assigned. For the two peaks with the highest s -values, these values (10.25 and 12.45 S) were consistent with those for the hydrodynamic parameters from the 3D reconstructions of ternary complex extended and compact conformations (9.55 and 11.95 S, respectively) [37] . These results support the existence of the extended and compact conformations for the Hsp90:Hop:Hsp70 complex. Structure of the ternary complex bound to a client protein To determine the next structural step in the Hsp70/Hsp90 folding pathway, that is, the formation of a quaternary Hsp90:Hop:Hsp70:substrate complex, we generated a complex between Hsp70 and the Hsp90-client protein GR-LBD (the ligand-binding domain of the glucocorticoid receptor) and incubated it with preformed Hsp90:Hop and ADP (no complex is formed with AMP-PNP) ( Supplementary Fig. 8a,b ). After EM, heterogeneity of the purified quaternary complex was similar to that of the ternary complex (compare Supplementary Fig. 8c and Fig. 5c ). We classified 32,618 particles by 2D methods to generate a homogeneous population, used for a 3D reconstruction and later refined by extensive 3D classification to generate a final 3D reconstruction of the compact structure (24 Å resolution; Fig. 7a ). This reconstruction was almost identical to that of the ternary complex, except for a small mass protruding from one of the long sides of the structure, in the Hsp90-M ( Fig. 7b ). 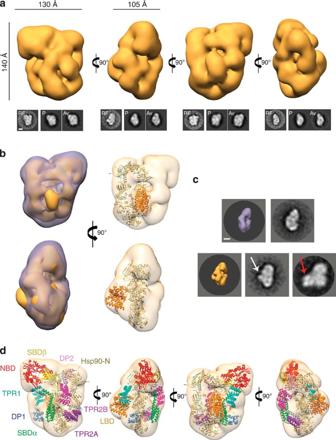Figure 7: 3D reconstruction of the Hsp90:Hop:Hsp70:GR-LBD complex. (a) Top, the four standard orthogonal views of the quaternary complex (24 Å resolution). Bottom, reference-free class averages (RF), projections (P) and 2D averages (Av) of the final model, shown in the same orientations as at the top. (b) Left, two orthogonal views of the Hsp90:Hop:Hsp70 complex 3D reconstructions (yellow, transparent) superimposed on the Hsp90:Hop:Hsp70:GR-LBD complex (orange, solid). Right, the same two views with the docking of the Hsp90 dimer (pdb 2IOP) and the GR-LBD (pdb 1M2Z) atomic structures. Scale bar, 50 Å. (c) Top, comparison of a lateral view of the Hsp90:Hop:Hsp70 complex with the 2D average view. Bottom, similar view of the Hsp90:Hop:Hsp70:GR-LBD complex (left) with the 2D average (centre) and the same view of an immunocomplex between the Hsp90:Hop:Hsp70GR-LBD complex and the anti-GR-LBD antibody (right). The white arrow indicates the position of the mass attributed to GR-LBD and the red, the mass attributed to the anti-GR:LBD antibody. (d) The same orthogonal views of the Hsp90:Hop:Hsp70:GR-LBD complex as inFig. 4i, with the atomic structures of Hsp90, the Hop domains TPR1, DP1, the TPR2A-TPR2B module and DP2, the Hsp70NBDand Hsp70SBDdomains and the GR-LBD atomic structure (pdb 1M2Z). Figure 7: 3D reconstruction of the Hsp90:Hop:Hsp70:GR-LBD complex. ( a ) Top, the four standard orthogonal views of the quaternary complex (24 Å resolution). Bottom, reference-free class averages (RF), projections (P) and 2D averages (Av) of the final model, shown in the same orientations as at the top. ( b ) Left, two orthogonal views of the Hsp90:Hop:Hsp70 complex 3D reconstructions (yellow, transparent) superimposed on the Hsp90:Hop:Hsp70:GR-LBD complex (orange, solid). Right, the same two views with the docking of the Hsp90 dimer (pdb 2IOP) and the GR-LBD (pdb 1M2Z) atomic structures. Scale bar, 50 Å. ( c ) Top, comparison of a lateral view of the Hsp90:Hop:Hsp70 complex with the 2D average view. Bottom, similar view of the Hsp90:Hop:Hsp70:GR-LBD complex (left) with the 2D average (centre) and the same view of an immunocomplex between the Hsp90:Hop:Hsp70GR-LBD complex and the anti-GR-LBD antibody (right). The white arrow indicates the position of the mass attributed to GR-LBD and the red, the mass attributed to the anti-GR:LBD antibody. ( d ) The same orthogonal views of the Hsp90:Hop:Hsp70:GR-LBD complex as in Fig. 4i , with the atomic structures of Hsp90, the Hop domains TPR1, DP1, the TPR2A-TPR2B module and DP2, the Hsp70 NBD and Hsp70 SBD domains and the GR-LBD atomic structure (pdb 1M2Z). Full size image We confirmed GR-LBD location by incubating the quaternary complex with an anti-GR-LBD antibody. We selected and classified 12,298 negatively stained particles; 2D analysis of the largest population showed a mass protruding from the same site at which GR-LBD was found in the 3D reconstruction ( Fig. 7c ). Docking of the GR-LBD [38] atomic structure into this extra mass of the reconstructed quaternary complex was good ( Fig. 7b ), as was the docking of all Hsp70 and Hop domains as assigned for the ternary complex ( Fig. 7d ). This suggests that GR-LBD bound to Hsp70 is delivered to one of two potential substrate-binding sites on the Hsp90 dimer, opposite the side where Hop is located. Hsp70 and Hsp90 are major chaperones in the protein folding pathway [39] . In the case of Hsp70, one of its functions is to assist Hsp90 in the maturation of specific proteins such as transcription factors, kinases and nuclear receptors. This process begins with Hsp70 recognition of the client protein, which is transferred to Hsp90 for subsequent folding or maturation [20] , [21] , [27] , [40] . This transfer is mediated by the co-chaperone Hop/Sti1, whereas the molecular basis of the Hsp90-Hop-Hsp70 interaction is well characterized [13] , [21] , there is little structural information about this process. Here we used low-resolution EM to determine the structure of the transient complexes in the Hsp70/Hsp90 pathway. Complexes were prepared by combining the appropriate partners; in all cases, after purification, we observed clear heterogeneity, which we consider inherent to these complexes. Part of this heterogeneity was overcome by the use of GraFix [29] , a method that has been successful with many complexes [41] , [42] and has helped to stabilize the most populated conformations. It is nonetheless clear that all three components are flexible, especially Hop, and that this flexibility is necessary for substrate transfer between the two chaperones. Although we used crosslinking, controls showed similar structural information for treated and untreated complexes (see Supplementary Fig. 4a ). The structures of the human and yeast Hsp90:Hop complexes in the presence of ADP ( Figs 1 and 2 , Supplementary Fig. 2 ) are similar and show the Hsp90 dimer in a semiclosed conformation, resembling that of the uncomplexed Hsp90 dimer ( Supplementary Fig. 5 ). Our structure differs from a recent 3D reconstruction of the human Hsp90:Hop complex, which showed an open conformation for the Hsp90 dimer without nucleotide [28] . This same semiclosed conformation is observed for the binary complex without crosslinker ( Supplementary Fig. 4a ) or molybdate, used to avoid Hsp90 proteolysis [43] ( Supplementary Fig. 4c ). In the case of Hop-free Hsp90, we also found other conformations, which suggests that Hop interaction restricts Hsp90 dimer flexibility [16] , [28] . The information reported so far indicates that the Hsp90 cycle has a multitude of conformations that depend on numerous factors (co-chaperones, client proteins, nucleotides) [6] , [9] , [44] , [45] ; other Hsp90:Hop complex conformations therefore cannot be ruled out. The 3D reconstructions of human and yeast Hsp90:Hop complexes indicate that a single Hop molecule interacts with the Hsp90 dimer, as confirmed by ultracentrifugation analysis ( Supplementary Fig. 7 ). These volumes differ from that published recently, showing a 2:2 (monomer:monomer) stoichiometry for Hsp90 and Hop [28] . At difference from these authors, we engineered no disulfide bridges between Hsp90 and Hop, the presence of which could force the binding of a second Hop molecule to the complex. Our immunomicroscopy experiments with specific antibodies and the use of Hop deletion mutants followed by docking of the Hop domains atomic structures, point to Hop interaction with one side of the Hsp90 dimer ( Fig. 2 , Supplementary Fig. 2 ). The five Hop domains are arranged in an anticlockwise fashion, such that TPR2A is in contact with Hsp90-C, its binding partner [19] , [46] , whereas TPR2B and DP2 interact mainly with Hsp90-M and Hsp90-N on one of the Hsp90 monomers [16] , [28] , [47] and TPR1-DP1 binds to similar regions on the other monomer. This last interaction appears to be weaker than the other two, as shown by the heterogeneity in this part of the structure, which has a percentage of the particles with a small mass protruding from the volume of the complex ( Supplementary Fig. 4b ). Release of the TPR1-DP1 module from the Hsp90:Hop complex core could allow Hsp90 and Hop interaction with other chaperones or co-chaperones, in accordance with other studies [14] , [27] . The arrangement of the Hop domains in the complex seems to prevent total closure of the Hsp90 dimer, thus blocking ATPase activity and generating a semiclosed conformation that allows client protein binding [16] , [27] , [28] . The human and yeast Hsp90:Hop:Hsp70 complexes were generated by incubating the three partners in the presence of Hsp40, which was not included in the final ternary complex, as reported elsewhere [21] ( Supplementary Fig. 6 ). Hsp40 interacts with Hsp70 through Hsp70 NBD , but also through the Hsp70 SBD C-terminal segment, in competition with Hop [48] , [49] , [50] . We suggest that Hsp40 interacts with Hsp70 and helps this chaperone to reach an appropriate conformation for Hop binding, after which is displaced by the co-chaperone. Our preparations of the human and yeast Hsp90:Hop:Hsp70 complex show two large populations that are better characterized by particle classification ( Fig. 5c ); the majority (~80%) has a compact shape and the other is extended (~15%). 3D reconstruction of the compact structure ( Figs 3 and 4 , Supplementary Fig. 6 ) shows a shape similar to that of the Hsp90:Hop complex, with the Hsp90 dimer in the same semiclosed conformation. The anticlockwise arrangement of Hop domains in the binary complex also fits well in this complex, which suggests there are no major changes for Hop domains after Hsp70 binding (see below). The major difference between the binary and ternary complexes resides in a mass that protrudes from Hsp90-N of one Hsp90 monomer, which we identified by immunomicroscopy as Hsp70 NBD . This domain is located in the Hsp90 monomer, opposite the monomer that interacts with the Hop TPR2A-TPR2B-DP2 module; this supports the idea of asymmetric interaction of the Hsp90 dimer with other chaperones and co-chaperones [14] , [16] , [27] . Once the interaction between Hsp70 and Hop takes place, there appears to be a further interaction between Hsp70 NBD and the Hsp90-N on one Hsp90 monomer, which stabilizes the compact conformation of the ternary complex [21] , [32] . This interaction is not stable on its own since there is no binding between purified Hsp70 NBD and Hsp90 (results not shown), but it takes place in the compact conformation of the ternary complex and cannot be explained by the crosslinking, since we found particles in which Hsp70 did not contact Hsp90 (the ‘extended’ complexes) and conversely, we found compact ternary complex structures in the crosslinker-free AUC experiments ( Supplementary Fig. 7 ). Nonetheless, Hsp70 and Hsp90 associate through Hop, via interactions between TPR2A and the C-terminal segment of one Hsp90 monomer on one side, and TPR1 or TPR2B and the Hsp70 C-terminal segment on the other [16] , [19] . According to these studies, Hsp70 SBD interacts first with TPR1, and is subsequently transferred to TPR2B. As our immunomicroscopy experiments with the compact conformation locate Hsp70 SBD near TPR1 and TPR2B ( Fig. 4 ), we cannot directly confirm or rebut the TPR1-TPR2B transfer of Hsp70 (but see below). Direct comparison of the binary and ternary complexes ( Fig. 5a,b ) nonetheless makes it clear that the presence of Hsp70 induces lateral movement of the Hop domains towards the Hsp70 molecule, which could have biological implications. Internalization of the active nucleus (TPR2A-TPR2B-DP2) after TPR1-DP1 module movement suggests that the linker between the two modules is responsible for allosteric control of Hop, which would thus contribute to the operation of the Hsp70/Hsp90 machinery. A recent study suggests that, thanks to the Hop flexibility, the Hsp90:Hop:Hsp70 complex switches between an extended conformation that recognizes and traps Hsp70 bound to a client protein, and a compact form in which the client protein is delivered to the Hsp90 dimer [16] . We reasoned that these two steps might be associated to the extended and compact conformations we observed by EM; these conformations might explain the absence of or decrease in client protein activation in Hop mutants that lack DP2 or have an altered TPR2B/Hsp70 interaction [16] , [51] , [52] , [53] . In the compact conformation, DP2 is located near Hsp70 SBD , and we suggest that the formation of the compact structure could have two roles. In the first step, Hsp70 would position the client protein in contact with DP2 for activation [16] , followed by Hsp70 SBD switching from TPR1 to TPR2B to induce the formation of the compact structure and release the client protein into the Hsp90-binding site. Study of the extended conformations was difficult, due to their small particle number and different degree of aperture. By extensive classification, we were able to reconstruct homogeneous populations of the extended conformations for the human ternary complex and for the yeast system using a Hop mutant (R469A). This altered Hop prevents Hsp70 binding to TPR2B [16] and was intended to favour the extended conformation. This was indeed the case, as the percentage of extended view particles was almost tripled (~40% in for the mutant yeast compared to ~15% for wild-type human ternary complex), which strengthens the idea that the Hsp70 SBD C-terminal segment interacts with TPR1 (in the extended conformation) or TPR2B (in the compact conformation). We used the docking established for the binary and compact ternary complexes to fit the various domains of the three partners into the extended structures, with the largest mass occupied by the Hsp90 dimer, the Hop TPR2A-TPR2B-DP2 module, TPR2B and DP2. The smaller mass was assigned to Hsp70 and the Hop domains TPR1 and DP1, whereas the linker was located between the DP1 and TPR2A domains in a non-structured region (~60 residues; Fig. 6b,d ). This docking is plausible and strengthens the concept of plasticity of Hop domains that, when bound to the Hsp90 dimer, search for Hsp70 (the Hsp70:client protein complex) and attract it to Hsp90 for subsequent interaction with this chaperone. The two 3D reconstructions of the extended conformation for the human and yeast systems are very similar, but differ in the degree of aperture of the two masses. We suggest that these two structures represent different steps in a complex that cycles between the extended and compact conformations ( Fig. 8a ). 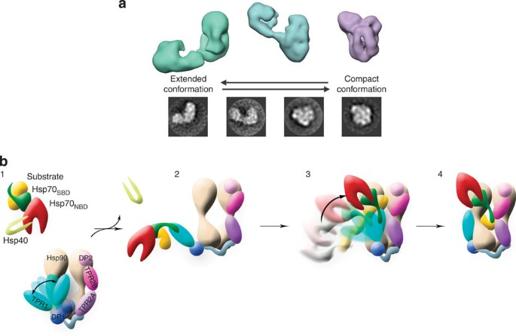Figure 8: Model of the Hop-mediated Hsp70/Hsp90-client protein transfer mechanism. (a) The Hsp90:Hop:Hsp70 complex cycles between an extended and a compact conformation. This is supported by the 3D reconstructions of the extended conformation of the human Hsp90:Hop:Hsp70 complex (left), that of the yeast Hsp90:Hop(R469A):Hsp70 complex (center), and the compact conformation of the human Hsp90:Hop:Hsp70 complex (right). Bottom, four reference-free classes observed in the total population of Hsp90:Hop:Hsp70 particles that also describe the movement between the extended and compact conformations. (b) Model of Hop-mediated substrate transfer between Hsp70 and Hsp90. (1) Hsp70 recognizes and traps an Hsp90-client protein through Hsp70SBDwith the help of Hsp40; interaction with this chaperone is transient. Hop and Hsp90 bind through the TPR2A and the C terminus of one Hsp90 monomer, respectively. There are other interactions between Hsp90 and Hop, although the co-chaperone shows considerable flexibility, in particular its TPR1 and DP1 domains, which cycle between a compact and an extended conformation. (2) The Hsp70:substrate complex and Hsp90:Hop interact through the C-terminal end of Hsp70SBDand the Hop TPR1 domain, respectively. (3) The movements described inainduce the approximation of the Hsp70:substrate:TPR1:DP1 and the Hsp90:TPR2A-TPR2B-DP2 parts of the Hsp90:Hop:Hsp70:substrate complex. (4) Hsp70 delivers the substrate to one of the two substrate-binding sites of the Hsp90 dimer, that opposite the Hop-binding site. Figure 8: Model of the Hop-mediated Hsp70/Hsp90-client protein transfer mechanism. ( a ) The Hsp90:Hop:Hsp70 complex cycles between an extended and a compact conformation. This is supported by the 3D reconstructions of the extended conformation of the human Hsp90:Hop:Hsp70 complex (left), that of the yeast Hsp90:Hop(R469A):Hsp70 complex (center), and the compact conformation of the human Hsp90:Hop:Hsp70 complex (right). Bottom, four reference-free classes observed in the total population of Hsp90:Hop:Hsp70 particles that also describe the movement between the extended and compact conformations. ( b ) Model of Hop-mediated substrate transfer between Hsp70 and Hsp90. (1) Hsp70 recognizes and traps an Hsp90-client protein through Hsp70 SBD with the help of Hsp40; interaction with this chaperone is transient. Hop and Hsp90 bind through the TPR2A and the C terminus of one Hsp90 monomer, respectively. There are other interactions between Hsp90 and Hop, although the co-chaperone shows considerable flexibility, in particular its TPR1 and DP1 domains, which cycle between a compact and an extended conformation. (2) The Hsp70:substrate complex and Hsp90:Hop interact through the C-terminal end of Hsp70 SBD and the Hop TPR1 domain, respectively. (3) The movements described in a induce the approximation of the Hsp70:substrate:TPR1:DP1 and the Hsp90:TPR2A-TPR2B-DP2 parts of the Hsp90:Hop:Hsp70:substrate complex. (4) Hsp70 delivers the substrate to one of the two substrate-binding sites of the Hsp90 dimer, that opposite the Hop-binding site. Full size image To visualize the final step in client protein transfer between chaperones Hsp70 and Hsp90, as well as its binding to the Hsp90 dimer, we prepared Hsp70:GR-LBD and Hsp90:Hop complexes and purified the quaternary complex ( Supplementary Fig. 8 ). The EM images show compact and extended structures that we associate with the presence of the Hsp90:Hop:Hsp70:GR-LBD complex in both conformations ( Supplementary Fig. 8c ). We focused on the majority, compact conformation and generated a volume almost identical to the ternary complex ( Fig. 7 ), except for a small mass protruding from Hsp90-M on one side of the Hsp90 dimer. The position of GR-LBD in this quaternary complex was confirmed by immunomicroscopy ( Fig. 7c ) at the same site at which this client protein was found in a Hsp90:GR-LBD complex [27] , the substrate-binding site of the Hsp90 dimer opposite the Hop location ( Fig. 7d ). Although the Hsp90 dimer hosts two identical binding sites for any given client protein, only one is available, as the other is occluded by the co-chaperone [27] , [54] . On the basis of these findings, we propose a structural model for Hop-mediated client protein transfer between Hsp70 and Hsp90 chaperones ( Fig. 8b ). First, (1) Hsp70 recognizes and binds an Hsp90-client protein through Hsp70 SBD . This is facilitated by Hsp40, which promotes a stable Hsp70:substrate complex by inducing the Hsp70 ADP, closed conformation. Hop in turn binds to the Hsp90 dimer and induces a semiclosed conformation, appropriate for subsequent client protein loading to Hsp90 (ref. 27 ). Hop and Hsp90 bind respectively via TPR2A and the C-terminal segment of one Hsp90 monomer. Next, (2) whereas the open Hsp90:Hop complex conformation traps the Hsp70:substrate complex through the Hop TPR1 domain and Hsp70 SBD , (3) the compact conformation places the Hsp70:substrate complex in contact with DP2 for client activation, and then with the Hsp90 dimer, through the movement of the TPR1-DP1 module. The client protein loads to the Hsp90 dimer through one of the two potential protein-binding sites that was not occluded by Hop. Finally, (4) before or after client protein delivery to Hsp90, Hsp70 interacts further with Hsp90, with Hsp70 NBD in contact with Hsp90-N on one of the Hsp90 monomers, whereas Hsp70 SBD is located near TPR2B [16] . This closer interaction between Hsp70 and Hsp90 induces lateral rearrangement of Hop domains, which we can only suggest is used for subsequent steps in the Hsp90-assisted folding pathway (for example, Hsp70 and Hop release, PPiase and p23 binding) [16] . Using EM and image processing, we isolated and 3D reconstructed several of the transient complexes formed during the protein maturation pathway assisted by the Hsp70 and Hsp90 chaperones and their co-chaperone Hop. This structural information provides the basis for improved molecular understanding of substrate transfer between these two chaperones and clarifies the first steps in the complex picture of the Hsp90 functional cycle, in which other co-chaperones are also involved. Protein expression and purification Human Hsp90α (hHsp90) cDNA was a generous gift of Dr J. Ávila (CBM-CSIC, Madrid) and was cloned into a pET-Duet1 vector (Novagen). Human Hsp70 (hHsp70), human Hsp40 (DNAJB1; hHsp40) and human Hop (hHop) cDNA were obtained from Source BioScience and were cloned into pQE-30UA (Qiagen), pET-24d(+) and pET-Duet1 (Novagen), respectively. All proteins were expressed in Escherichia coli Rosetta strain. hHsp90, hHsp70 and hHsp40 proteins (all with a 6xHisTag, in the N (Hsp90, Hsp70) or the C terminus (Hsp40)). Proteins from bacterial lysates were purified by Ni-NTA affinity column chromatography (GE Healthcare), followed by gel filtration chromatography (Superdex 200 column, GE Healthcare). hHop from the bacterial lysate was purified by two ion exchange chromatography steps (Heparin and Q-Sepharose, GE Healthcare), followed by gel filtration (Superdex 200). The yeast proteins Ssa1 (yHsp70), Sti1 (yHop), Sti1(R469A), yHsp90, Ydj1 (yHsp40) were expressed and purified [16] , [27] , [55] , [56] . The stabilized GR mutant (GR-LBD; F602S/A605V/V702A/E705G/M752T) was expressed and purified [27] . Δ(TPR1-DP1)Hop, a mutant lacking the TPR1 and DP1 domains (1–224 region), was constructed in the pCold I vector (Takara, Tokyo, Japan), which contains 6xHisTag in the N terminus, and expressed and purified [57] . The Fab fragment of the Hsp70 SBD antibody was generated with the Mouse IgG1 Fab and F(ab′) 2 Kit (Thermo Scientific). In vitro assembly and purification of Hsp90 complexes Hsp90:Hop and Hsp90:Δ(TPR1-DP1)Hop complexes were formed by incubating appropriate proteins (hHsp90, hHop and Δ(TPR1-DP1)Hop, respectively, Supplementary Table I ) in binding buffer C (20 mM HEPES pH 7.5, 50 mM KCl, 1 mM diothiothreitol, 5 mM MgCl 2 and 5 mM ADP) at 35 °C for 40 min. Samples were then incubated with 20 mM sodium molybdate (35 °C, 5 min) to avoid autoproteolysis and to stabilize the complexes [43] , [58] , and then loaded onto a Superdex 200 column equilibrated in buffer GF (20 mM HEPES pH 7.5, 50 mM KCl, 1 mM diothiothreitol, 5 mM MgCl 2 and 1 mM ADP). Aliquots of fractions from the same gel filtration experiment were chemically crosslinked with 0.005% glutaraldehyde [59] . Fractions alone or with glutaraldehyde were analysed by SDS-polyacrylamide gel electrophoresis. Complexes and immunocomplexes (antibodies used: mAb-Hsp70 NBD , mAb-Hsp70 αSBD (both from Enzo Life Science), mAb-Hop (DP2) (Abgent), pAb-GR (LBD) (Acris Antibodies) were formed by incubation in binding buffer C (35 °C, 40 min) for the human proteins and 28 °C for yeast proteins ( Supplementary Table I ). Sodium molybdate (20 mM) was added to complexes, which were then purified using GraFix in buffer GF [29] . Complexes and immunocomplexes generated using Fab fragments were purified in a glycerol/glutaraldehyde gradient (10–30%/0–0.15%, respectively) at 32,000 r.p.m. in a SW 55 Ti rotor (Beckman-Coulter)(16 h, 4 °C). Immunocomplexes with full-length antibodies were purified in a glycerol/glutaraldehyde gradient (10–40%/0–0.15%, respectively) (32,000 r.p.m., 16 h, 4 °C). Mobility controls of individual proteins and complexes without glutaraldehyde gradient were carried out in the same conditions. Gradients were fractionated in 200 μl samples and analysed by SDS-polyacrylamide gel electrophoresis and silver stain. EM and image processing Aliquots of Hsp90 or the various Hsp90 complexes were applied to glow-discharged carbon grids (7 min), washed and stained with 2% (w/v) uranyl acetate (1 min). Micrographs were recorded in a JEOL 1200EX-II electron microscope, operated at 100 kV, on Kodak SO-163 film at 60,000 nominal magnification. Micrographs were digitized in a Zeiss SCAI scanner to a final sampling resolution of 2.33 Å per pixel. Individual particles were selected manually using the software package XMIPP [60] . Initial analysis of the data and two-dimensional classification using maximum-likelihood procedures were carried out as described [61] . Representative averaged 2D images to a comparative analysis were obtained using KerdenSOM [62] . For 3D analysis, the particles were processed by angular refinement techniques implemented in EMAN [63] . To avoid model bias, several models (including blob, common lines, noise) were used as starting volumes for refinement and in all cases the volumes evolved toward a common 3D solution (see Supplementary Fig. 3 ). No symmetry was assumed for any of the refinements. Several rounds of 3D classification were performed using three-dimensional maximum-likelihood techniques [64] due to sample heterogeneity and the most consistent volume was used for new refinement rounds. Projection-matching protocols implemented in XMIPP were used for final refinement. Resolution was estimated with Fourier shell correlation using the 0.5 correlation coefficient criteria [65] . Docking of the atomic structure of related proteins into 3D reconstructions was carried out manually and optimized using USCF Chimera [66] . Analytical ultracentrifugation experiments Sedimentation velocity analyses of the individual components (Hsp90, Hop, Hsp70) or the complexes (Hsp90:Hop and Hsp90:Hop:Hsp70) were carried out in the absence of crosslinker in an Optima XL-I analytical ultracentrifuge (Beckman-Coulter). All experiments were performed at 185,000 g and 20 °C. Complexes were detected by ultraviolet–visible absorbance and Raleigh interference optics. Differential sedimentation coefficient distributions ( c(s) ) were calculated by least squares boundary modelling of sedimentation velocity data using the programme SEDFIT [67] , [68] . From this analysis, the experimental sedimentation coefficients were corrected for solvent composition with the programme SEDNTERP [69] to obtain the standard s -values. Experimental values for Hsp90 and the binary and ternary complexes were then correlated with the theoretical s -values obtained from the EM 3D structures, using HYDROMIC [37] . How to cite this article: Alvira, S. et al . Structural characterization of the substrate transfer mechanism in Hsp70/Hsp90 folding machinery mediated by Hop. Nat. Commun. 5:5484 doi: 10.1038/ncomms6484 (2014).